Primate evolution of the recombination regulator PRDM9 The PRDM9 gene encodes a protein with a highly variable tandem-repeat zinc finger (ZF) DNA-binding domain that plays a key role in determining sequence-specific hotspots of meiotic recombination genome wide. Here we survey the diversity of the PRDM9 ZF domain by sequencing this region in 64 primates from 18 species, revealing 68 unique alleles across all groups. We report ubiquitous positive selection at nucleotide positions corresponding to DNA contact residues and the expansion of ZFs within clades, which confirms the rapid evolution of the ZF domain throughout the primate lineage. Alignment of Neandertal and Denisovan sequences suggests that PRDM9 in archaic hominins was closely related to present-day human alleles that are rare and specific to African populations. In the context of its role in reproduction, our results are consistent with variation in PRDM9 contributing to speciation events in primates. Genes that cause hybrid sterility between species have the potential to reveal important insights into reproduction and the evolutionary mechanisms that drive speciation [1] . PRDM9 , a gene involved in meiotic recombination that was identified as a hybrid sterility gene in mammals [1] , [2] , [3] , [4] , encodes a protein with a KRAB domain, a PR/SET histone H3(K4) trimethyltransferase domain and a DNA-binding domain consisting of a variably sized tandem-repeat array of C 2 H 2 zinc fingers (ZFs) [2] ( Fig. 1 ). PRDM9 is active during meiosis I and regulates recombination events by marking DNA for double-strand breaks at locations targeted by the ZF domain [5] , [6] . High levels of genetic diversity in the ZF domain have been observed within and between species [7] , and this diversity has been suggested as a source of variation in recombination hotspot motifs between taxa [2] . The observation that variation in the PRDM9 gene may lead to sterility in human males [8] and hybrid sterility in mice [1] has fueled speculation that the gene can cause post-zygotic reproductive isolation in otherwise closely related individuals, ultimately leading to speciation events [7] . 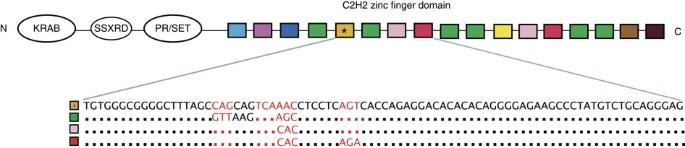Figure 1: Schematic representation of thePRDM9gene. The C2H2ZF domain consists of a variably sized array of ZF repeats, which are represented as differentially coloured boxes (allele Pan.t-1 diagrammed here). Each array possesses many distinct ZFs, with some repeating at multiple positions throughout the array. The nucleotide sequence of four internal fingers is shown, and identical codons from different fingers are represented as dots. The high sequence similarity between different fingers demonstrates the repetitive nature of the ZF array. The nucleotide positions that code for the protein’s DNA contact loci are coloured in red. Figure 1: Schematic representation of the PRDM9 gene. The C 2 H 2 ZF domain consists of a variably sized array of ZF repeats, which are represented as differentially coloured boxes (allele Pan.t-1 diagrammed here). Each array possesses many distinct ZFs, with some repeating at multiple positions throughout the array. The nucleotide sequence of four internal fingers is shown, and identical codons from different fingers are represented as dots. The high sequence similarity between different fingers demonstrates the repetitive nature of the ZF array. The nucleotide positions that code for the protein’s DNA contact loci are coloured in red. Full size image To further investigate the potential role of PRDM9 in primate evolution, we sequenced the ZF array in a diverse set of primates and re-analysed reads corresponding to this locus in published genomes from Neandertal and Denisovan individuals. Rapid evolution of the PRDM9 gene was seen across all primates, presumably resulting in distinct recombination landscapes for each species, and novel ZFs were found in the ancient hominins. These findings confirm that PRDM9 diversity is found throughout the primate lineage and provide further support to the idea that PRDM9 plays a role in primate speciation. Sequencing of the PRDM9 ZF array We surveyed the genetic diversity contained within the hypervariable ZF domain of PRDM9 in 64 individuals from the following genera: Pan , Homo , Gorilla , Pongo , Hylobates , Symphalangus , Nasalis , Papio , Macaca , Simia and Callithrix ( Supplementary Tables 1 and 2 ). Because of the length and highly repetitive nature of the PRDM9 ZF array, we used bacterial cloning, nested Sanger sequencing and manual curation of reads into full-length assemblies of individual alleles (we use the term ‘allele’ here to refer the full-length, nucleotide-level sequences of ZF arrays, and consider alleles to be unique if they differ at the nucleotide level). Before this study, two other groups characterized 21 non-hominid ZFs across 25 alleles within the Pan genus [9] , [10] . Here we report an additional 148 ZFs from 40 previously uncharacterized alleles across 11 primate genera ( Supplementary Data 1 ). Identical protein sequences for single ZFs were shared between individuals from different genera in only seven instances ( Supplementary Fig. 1 ). There were three instances of ZF arrays identical at the protein level between individuals from different species (Gor.g-4 in Gorilla beringei and Gorilla gorilla ; Hyl.p-1 in Hylobates pileatus and Hylobates gabriellae ; and Pan.p-1 in Pan paniscus and Pan.t-6 in Pan troglodytes ), two of which (the Gorilla and Hylobates pairs) were also identical at the nucleotide level, that is, identical alleles as per our terminology ( Supplementary Table 3 ). 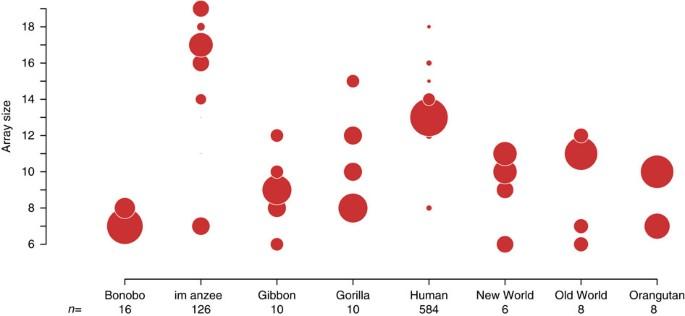Figure 3: Diversity inPRDM9ZF array size. The size of each circle is proportional to the abundance of alleles of a given array size within the labelled taxonomic grouping. The ‘n’ value is the number of alleles sampled for each group. Only those individuals that had both alleles characterized were included. Evidence for positive selection The DNA-binding specificity of PRDM9 is determined by the residues at positions −1, 2, 3 and 6 of each ZF, and these positions show strong signals of positive selection in humans [11] and chimpanzees [10] . To explore whether positive selection is acting on these residues in other primate lineages, we performed a pairwise codon alignment of ZFs within each genus and generated Bayes–Emperical–Bayes d N /d S estimates. We found overwhelming evidence for positive selection at positions −1, 3 and 6 across all genera, and at position 2 in some genera. There was also evidence for positive selection at positions not in contact with DNA ( Fig. 2 ). In addition to the ZF diversity, the size of the arrays was highly variable, with a range from 6 to 19 across all species ( Fig. 3 ). 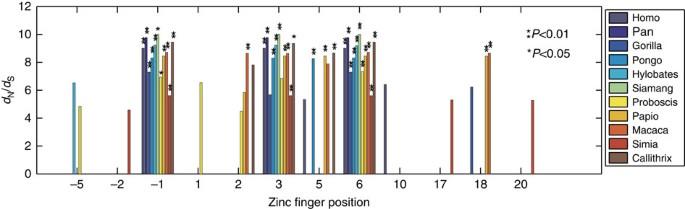In mice, it has been shown that PRDM9 arrays differing in size by a single finger can lead to hybrid sterility [1] , but given the highly heterogeneous size of ZF arrays within the species examined here, this seems unlikely to generalize. Figure 2: Evidence for positive selection acrossPRDM9ZFs in primates. Bayes–Empirical–BayesdN/dSestimates at ZF positions for which there exists evidence of positive selection are shown. Almost all genera showed strong positive selection at DNA contact positions (−1, 3 and/or 6) with the Bonferroni correction method for multiple testing. Figure 2: Evidence for positive selection across PRDM9 ZFs in primates. Bayes–Empirical–Bayes d N /d S estimates at ZF positions for which there exists evidence of positive selection are shown. Almost all genera showed strong positive selection at DNA contact positions (−1, 3 and/or 6) with the Bonferroni correction method for multiple testing. Full size image Figure 3: Diversity in PRDM9 ZF array size. The size of each circle is proportional to the abundance of alleles of a given array size within the labelled taxonomic grouping. The ‘ n ’ value is the number of alleles sampled for each group. Only those individuals that had both alleles characterized were included. Full size image ZF binding predictions We generated predicted binding motifs for the 15 most common chimpanzee alleles (Pan.t-1 to Pan.t-15, each seen in at least two individuals) and all of the other primate alleles [12] ( Supplementary Fig. 2 ). The allele repertoire for each species is predicted to bind distinct motifs with little to no overlap between species. Although there is substantial binding site diversity within the most frequent chimpanzee alleles, we found that there is a short common motif shared by many of them (AATTnnAnTCnTCC). 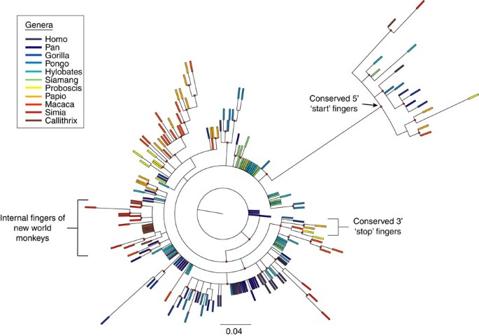Figure 4: Phylogenetic tree demonstrating evolutionary relationships between ZFs. Maximum-likelihood reconstruction of the ZF phylogeny, coloured by genus. Each finger is represented with a coloured bar and branches with strong approximate likelihood ratio test (aLRT) values (>0.8) are marked with red circles. The most 5′ fingers from all genera form a clear clade with an aLRT value of 1. The most 3′ ‘stop’ fingers are also closely related (aLRT value 0.86) in several distantly related genera. In contrast, intra-species similarity can be seen throughout the rest of the tree, where fingers from the same or closely related genera form clusters, consistent with a concerted evolution mechanism. This is most clearly exhibited in the New World monkeys, where nearly all internal fingers are very closely related to one another, especially in theCallithrix jacchus(brown bars). We investigated whether this motif has undergone any substantial depletion specifically within the chimpanzee lineage, but found it to be equally prevalent in the human, chimpanzee and gorilla genomes [13] ( Supplementary Table 4 ). However, it should be emphasized that there is considerable uncertainty in computational motif prediction for large ZF arrays, and performing experimental binding assays may be critical for defining the actual motifs and possible recombination hotspots specified by these alleles. Evolutionary dynamics of primate PRDM9 ZF arrays The fact that PRDM9 fingers display greater sequence identity within species than between species is consistent with observations in other tandem satellite families, and is evidence that the PRDM9 ZF locus is undergoing concerted evolution [14] . To further investigate the evolutionary dynamics of the PRDM9 ZF domain, we constructed a maximum-likelihood tree using an alignment of all primate ZF DNA sequences with codons encoding contact residues masked because of their extreme diversity ( Fig. 4 ). Statistical support is low for many branches, but we nonetheless observe clear structure within parts of the phylogeny. Remarkably, all of the 5′-most fingers in the ZF array form a well-defined, strongly supported clade, suggesting that an ancestral finger has retained this position throughout the primate lineage. At the 3′-most position, a distinct ancestral finger appears to have retained its position in old world monkeys, gibbons and Sumatran orangutans, but has been displaced by internal fingers in other species ( Fig. 4 and Supplementary Fig. 1 ). The dynamics at internal finger positions are clearly much more complex, but some interesting patterns can be discerned. For example, the ZFs in New World monkeys, especially Callithrix jacchus , cluster very tightly together on the tree, suggesting that a single ancestral ZF expanded to all but the 5′-most position of the ZF array along this lineage. The patterns and extent of diversity we observe at PRDM9 are consistent with the germline instability of the ZF domain shown by Jeffreys et al. [15] , although it remains unclear whether the apparently higher constraints on the 5′- and 3′-most ZF positions are a consequence of selection or mutational mechanism. Overall, the remarkable diversity observed in the ZF domain across 11 primate genera suggests that PRDM9 may activate recombination hotspots that are largely unique to each primate species, consistent with the lack of conservation in hotspot usage between chimpanzees and humans [9] , [16] . Figure 4: Phylogenetic tree demonstrating evolutionary relationships between ZFs. Maximum-likelihood reconstruction of the ZF phylogeny, coloured by genus. Each finger is represented with a coloured bar and branches with strong approximate likelihood ratio test (aLRT) values (>0.8) are marked with red circles. The most 5′ fingers from all genera form a clear clade with an aLRT value of 1. The most 3′ ‘stop’ fingers are also closely related (aLRT value 0.86) in several distantly related genera. In contrast, intra-species similarity can be seen throughout the rest of the tree, where fingers from the same or closely related genera form clusters, consistent with a concerted evolution mechanism. This is most clearly exhibited in the New World monkeys, where nearly all internal fingers are very closely related to one another, especially in the Callithrix jacchus (brown bars). Full size image Chimpanzee PRDM9 diversity and population structure To explore the diversity of the ZF locus within a single species, we combined the results from two previous chimpanzee-sequencing studies [9] , [10] with the large cohort in our study. The resulting data set consisted of 79 individuals with 142 chromosomes characterized (16 individuals were missing data for one allele) ( Supplementary Table 2 ). In total, we documented 34 alleles comprising varying combinations of 23 ZFs ( Fig. 5 ). Of the 63 individuals with data for both chromosomes, 67% (42/63) were heterozygous, and there were 45 different genotypes with only 11 genotypes present in multiple individuals. To test for Hardy–Weinberg equilibrium, we organized the alleles into three distinct groups according to 5′-structural similarity ( Fig. 5 ). Interestingly, the population is not at equilibrium when analysed in this way, with group ‘B’ allele homozygotes at a higher prevalence than expected ( χ 2 -test P -value <0.001). Consistent with population stratification as an underlying explanation, in the Groeneveld et al. [10] and Auton et al. [9] studies, all individuals with a ‘B’ group allele belonged to chimpanzee subspecies Pan troglodytes troglodytes or Pan troglodytes schweinfurthii (subspecies data was unavailable for individuals sequenced in our study). These two subspecies form a monophyletic clade within Pan troglodytes [17] , suggesting that some PRDM9 alleles possibly arose within certain chimpanzee lineages, and providing further support that the gene is undergoing concerted evolution in primates. 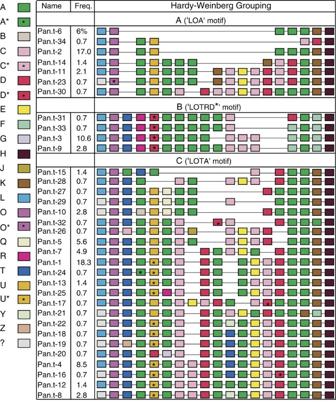Figure 5:PRDM9ZF array diversity in chimpanzees. Shown is a schematic representation of the ZF arrays of the 34 chimpanzee alleles described across three data sets. Each coloured box represents a different finger, and asterisks denote fingers with synonymous differences. The grey boxes represent fingers that were not sequenced but are assumed to be ZF ‘L’. The variability in ZF content and array size can be clearly seen in the different alleles. Although the rapid evolution of the ZF domain structure makes it difficult to precisely detail ancestral relationships between alleles, the 5′-end of the arrays displays structural patterns that enable alleles to be grouped for Hardy–Weinberg analysis. Figure 5: PRDM9 ZF array diversity in chimpanzees. Shown is a schematic representation of the ZF arrays of the 34 chimpanzee alleles described across three data sets. Each coloured box represents a different finger, and asterisks denote fingers with synonymous differences. The grey boxes represent fingers that were not sequenced but are assumed to be ZF ‘L’. The variability in ZF content and array size can be clearly seen in the different alleles. Although the rapid evolution of the ZF domain structure makes it difficult to precisely detail ancestral relationships between alleles, the 5′-end of the arrays displays structural patterns that enable alleles to be grouped for Hardy–Weinberg analysis. Full size image We sequenced too few primates to perform comparable analyses in other taxa, but in a separate study conducted in humans [18] , 25 unique PRDM9 alleles were described in a cohort of 124 individuals (248 chromosomes) of both European and African descent. There were 36 distinct genotypes and 51% (63/124) of individuals were heterozygous, and the most common allele in humans was at a much higher prevalence than the most common chimpanzee allele (68.5% versus 18.3%) ( Supplementary Fig. 3 and Supplementary Table 5 ). Some human alleles are only present in either the European or African lineage, demonstrating PRDM9 population stratification in humans as well ( Supplementary Table 5 ). We anticipate that more extensive sequencing of other primate genera will continue to reveal PRDM9 diversity as a reflection of the underlying population structure within each species. Polymorphism informational content (PIC) values are a useful determinant of the diversity present at a given locus [19] . We calculated [12] , [20] the PIC value for our chimpanzee cohort to be 0.9, while in humans it was only 0.51. For reference, one of the most diverse gene in humans [21] , HLA-B , was shown in one study of 234 individuals (436 chromosomes) to have a PIC value of 0.95 (ref. 22 ). The fact that PRDM9 is so much more diverse in chimpanzees, approaching the level of diversity seen in the most diverse human gene, is perhaps unsurprising given that Pan troglodytes is known to be more genetically diverse than humans, but whether this increased diversity at the PRDM9 ZF locus is a reflection of population history or biological constraint is difficult to assess [17] . Characterization of PRDM9 ZFs in ancient hominins To explore the more recent evolution of PRDM9 , we mapped the raw sequence reads from the high-coverage Neandertal [23] and Denisovan [24] genome projects to a library of all known primate adjacent finger pairings. Although Neandertals, Denisovans and modern humans diverged between 381,000 and 473,000 years ago [14] , we found that they share both PRDM9 ZF sequences and ZF linkages ( Fig. 6 and Supplementary Figs 4 and 5 ). The Denisovans, however, have two ZFs with synonymous changes that appear to be unique to their lineage, as they have not been observed in humans. Furthermore, two adjacent finger pairings that are rare and specific to modern African populations [18] were observed in the Denisovan and Neandertal shotgun data: D–R and D–S (finger–finger nomenclature adopted from Berg et al. [18] ; minor allele frequencies within African populations are 0.025 and 0.008, respectively). 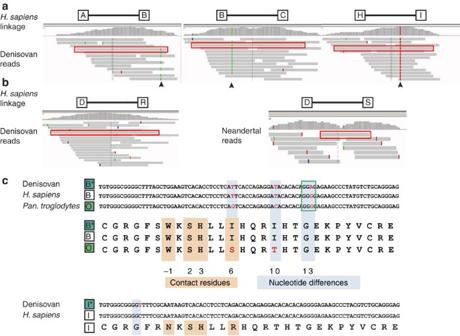Figure 6: PRDM9 ZF profile of early hominins. Raw reads from the Denisovan and Neandertal genome projects were mapped against primatePRDM9ZF linkages. (a) For three of the human linkages, we identified positions that had changed along the Denisovan lineage (marked with an arrow), which we denote as new fingers B* and I* (synonymous to human fingers B and I, respectively). Reads encompassed by a red box sufficiently span the exclusively identifying positions of both fingers to identify a finger–finger linkage. Note that not all mapped reads are shown. (b) Two rare human linkages, D–R and D–S, were only identified in the raw Denisovan and Neandertal datasets, respectively. (c) Codon alignments for the two new Denisovan fingers. For the B* finger (top), a synonymous change (G→A) at position 13 is unique to the Denisovan lineage, whereas both humans and chimpanzees have the ancestral base (G). For the I* finger (bottom), the Denisovan finger contains a derived synonymous change at position -4 (C→T). Figure 6: PRDM9 ZF profile of early hominins. Raw reads from the Denisovan and Neandertal genome projects were mapped against primate PRDM9 ZF linkages. ( a ) For three of the human linkages, we identified positions that had changed along the Denisovan lineage (marked with an arrow), which we denote as new fingers B* and I* (synonymous to human fingers B and I, respectively). Reads encompassed by a red box sufficiently span the exclusively identifying positions of both fingers to identify a finger–finger linkage. Note that not all mapped reads are shown. ( b ) Two rare human linkages, D–R and D–S, were only identified in the raw Denisovan and Neandertal datasets, respectively. ( c ) Codon alignments for the two new Denisovan fingers. For the B* finger (top), a synonymous change (G→A) at position 13 is unique to the Denisovan lineage, whereas both humans and chimpanzees have the ancestral base (G). For the I* finger (bottom), the Denisovan finger contains a derived synonymous change at position -4 (C→T). Full size image Diversity of PRDM9 outside of the ZF locus Recent work [15] suggests that PRDM9 may actually influence the instability of its own coding sequence in humans, and that rapid remodelling of alleles predicts fast changes in hotspot usage. To determine whether the region of genomic instability is restricted to PRDM9 ’s ZF region or whether it extends into surrounding genomic sequence, we used long-range PCR and massively parallel sequencing to explore nearby variation in a subset of primates. We found that the region immediately flanking the ZF region (3.2 kb on the 5′-end and 1.4 kb on the 3′-end) contained approximately the expected number of homozygous differences relative to the human genome [17] ( Supplementary Fig. 6 , Supplementary Table 6 and Supplementary Data 2–20 ). Variation in these immediately flanking regions enables accurate reconstruction of a species-level phylogeny for all great apes ( Supplementary Fig. 7 ), consistent with the markedly elevated genetic diversity being restricted to the ZF array alone and the absence of any deep coalescence as is the case at other highly polymorphic loci such as the major histocompatibility complex locus. In summary, we report the first large-scale survey of the genetic diversity of PRDM9 across the primate lineage. The remarkable amount of genetic diversity present between otherwise closely related species demonstrates that this gene is rapidly evolving in all or nearly all primates. Furthermore, the high levels of positive selection at the DNA contact positions and extensive structural variation with the ZF array suggest that these alleles are probably functional and active in specifying hotspot locations. Taken together, our data are consistent with the idea that variation in PRDM9 can lead to differential hotspot usage, which may result in hybrid sterility and contribute to speciation in the primate lineage. High-throughput functional testing of these different PRDM9 alleles is needed to identify their cognate DNA-binding sites, and phased genome sequencing of corresponding primate genomes may facilitate mapping of recombination hotspots. It is likely to be that we have only begun to sample the extent of the genetic diversity present in the PRDM9 gene in primates, and that continued exploration of its functional consequences will yield further insight into mechanisms that drive evolution and speciation events. Amplification and sequencing of the ZF PRDM9 array Primate genomic DNA was obtained from the Coriell Cell Repositories or Evan Eichler’s Lab at the University of Washington ( Supplementary Table 1 ). In the preliminary phase of this study, we tested out multiple different primer pairs in combination with a high-fidelity and long-processivity DNA polymerase on four chimpanzee individuals ( Supplementary Table 7 : ‘Pilot set of primers’). The aim of this phase was to discover an optimal set of primer sequences, PCR conditions and size-selection procedures to maximize product while minimizing chimera formation and nonspecific amplification of the PRDM9 homologue PRDM7. PCR and sequencing primers were designed using Primer3 to selectively amplify the ZF region of PRDM9 based on the chimpanzee reference genome (chr5: 91,796,444–91,798,315, CSAC 2.1.4/panTro4, Supplementary Table 7 ). We identified a subset of optimal primers that included >50 bp of unique, non-repetitive flanking sequence around the ZF array ( Supplementary Table 7 : ZF_forward, ZF_reverse, Mac_ZF_f, Mac_ZF_r) to use with the entire primate sample set. Real-time PCR was performed on 10 ng of genomic DNA using Kapa HiFi HotStart ReadyMix with the following thermal cycling protocol: 95 °C for 180 s, repeat (98 °C for 20 s, 65 °C for 15 s, 72 °C for 80 s). Each reaction was stopped before it left the exponential amplification stage to minimize PCR artefacts (for example, chimeras), which tend to amplify preferentially in the post-exponential amplification phase. Products were size-separated and size-selected using polyacrylamide gel electrophoresis (PAGE, for example, gel image in Supplementary Fig. 8 ). Chimeras, PRDM7 and primer–primer dimers were typically seen as fainter ladder-like bands beneath the main band when analysed via PAGE. To improve our specificity for sequencing PRDM9 , the largest and brightest bands corresponding to full-length amplification were size-selected from the gel. This procedure also allowed us to isolate and sequence arrays that differed in size by as little as one finger (84 bp). Size-selected products were cloned into pUC19 (InFusion, Invitrogen), transformed into Escherichia coli NovaBlue competent cells (EMD Millipore) and 4–24 single colonies for each PCR product were picked by hand for amplification by TempliPhi (GE Healthcare Life Sciences). Selecting multiple clones minimized the false-positive rate of any rare chimeric product that had the same size as a true allele. Without additional purification, clonally amplified DNA was Sanger sequenced at GENEWIZ using four different sequencing primers giving 900–1,000 bp of sequence in the forward and reverse directions ( Supplementary Table 7 : Sanger_F, Sanger_R, M13F, M13R). In total for the 64 primates studied, we sequenced 723 unique clones each with ≥2 different primer combinations in 2,270 independent Sanger-sequencing reactions (not all clone:primer combinations were attempted). See Supplementary Table 2 for the number of clones, primer pairs and reads analysed for each sample. Forward and reverse reads that had sufficient overlap (typically ≥2 unique fingers) were used to stitch together a consensus sequence for each clone ( Supplementary Table 3 and Supplementary Data 1 ). To be considered a valid sequence, at least two clones had to have identical sequence supporting a given consensus sequence. If only one band was present on PAGE and all clones generated from the isolated DNA had identical sequence, the individual was considered homozygous. Any aberrant sequences that differed from the canonical finger structure were discarded, and when necessary, samples were re-amplified and sequenced. All sequence data was visualized in Sequencher (Gene Codes Corporation). Identification of new PRDM9 fingers in Neandertal and Denisova shotgun data The raw sequence data for the Altai Neandertal and Denisova genomes was downloaded from the Max Planck Institute for Evolutionary Anthropology. First, we mapped all reads using mrsFAST [25] to a reference library comprising all known primate PRDM9 nucleotide sequences, allowing for an edit distance of up to 3. This revealed that the vast majority of mapped reads were either perfect matches or had a single base change with respect to a human PRDM9 sequence ( Supplementary Fig. 4 ). Given the highly repetitive nature of the ZF region and the short-read nature of the data, many reads did not exclusively identify a linkage or even a finger. However, there were enough longer reads that spanned through an exclusively identifying region of two fingers to prove informative. We refer to a ‘linkage’ as a unique combination of any two primate ZF sequences. A read will identify the presence of a linkage if it spans both the junction and the exclusively identifying variants in both fingers. We wanted to identify two things: (1) the presence of known primate linkages and (2) the presence of novel fingers/linkages. First, we generated a reference consisting of all known 168 bp primate PRDM9 ZF linkages (that is, Homo A–B, B–C, C–D and so on). For each linkage, we identified all the reads that mapped to it exclusively and perfectly without error. These reads were then removed from the mapped position file so that they would not inadvertently indicate the presence of variants in other linkages. By repeating this process for every linkage, the list of reads was effectively divided into two groups: those that map perfectly and exclusively to a linkage and those that map to a linkage but are either not exclusive or differ at one or more positions (we call this group the uncertain origin group (UOG)). To identify novel fingers or linkages, one by one we merged each linkage’s exclusive and perfect reads and all of the UOG reads and re-mapped them together. This effectively gives all the UOG reads a chance to vote for their presence in each linkage, while allowing the perfect and exclusive reads to vote only for their perfect linkages. After repeating this process for all known linkages, novel fingers were identified through manual curation of the resulting pileups ( Fig. 6a ). We used Monte Carlo simulations to identify the minimum possible set of PRDM9 linkages that still accurately represented the available data. We started by mapping all reads to the collection of all possible linkages (including all possible linkages involving the newly discovered fingers B* and I*) and counting the number of perfectly mapped reads ( Supplementary Fig. 5 ). Next, we randomly deleted one of the linkages in the reference library and re-mapped the reads. If the number of perfectly mapped reads remained unchanged, the process was repeated: another linkage was randomly deleted from the reference and the reads were re-mapped again. If there were fewer mapped reads after deleting a linkage, the linkage was returned to the library and the process was repeated. This cycle was repeated until a reduced set of core linkages was obtained, identified at the point whereby deleting any of them would result in additional reads that do not perfectly map. Owing to the nature of this random walk through linkage space, not all linkages present in the final set are necessarily unique. Some may instead represent one out of a few equally possible alternatives. To identify these uncertain linkages, we repeated the entire simulation at least ten times and kept track of which linkages appeared at the end of every simulation. Such linkages that appeared at the end of every trial were deemed to be necessary; that is, the data cannot be reconciled unless they are present. Amplification and sequencing of the PRDM9 flanking genomic sequence Real-time PCR was performed as described above using Kapa HiFi HotStart ReadyMix as directed by the manufacturer ( Supplementary Table 7 : 5.8 kb_forward/reverse, 5.8 kb_f_alt/r_alt), depending on the desired target, and the following thermal cycling protocol: 95 °C for 180 s, repeat (98 °C for 20 s, 65 °C for 15 s, 72 °C for 180 s). Samples were loaded on a 1% agarose gel and run for 1 h at 100 V. Bands of the desired size were size selected and purified ( Supplementary Fig. 9 ). A four-fold larger volume PCR using the same conditions was then run using the size-selected sample as the template. The PCR products were pooled for each individual and purified using Agencourt AMPure magnetic beads, following the manufacturer’s protocol. Samples were eluted in 50 μl and loaded directly into the Covaris Adaptive Focused Acoustics machine. Standard shotgun libraries were then prepared for paired-end (2 × 250 bp) Illumina MiSeq sequencing (sequencing primers in Supplementary Table 7 : MiSeq_p7 and MiSeq_p5). Tests for positive selection To detect sites under positive selection, we performed a multiple sequence alignment of all ZF DNA sequences for each genus (Clustal Omega) [26] . The phylogenetic guide trees generated were then used as input to test for positive selection using the codeml package of PAML v4.7 (ref. 27 ) as previously described, with the Bonferroni correction for multiple testing. ZF array binding site prediction We used the methods described by Persikov et al. [12] to generate predicted binding motifs for the 15 most frequent chimpanzee alleles (Pan.t-1 to Pan.t-15, each seen in at least two individuals) and all of the other primate alleles. Briefly, each ZF array was translated into amino acid sequence and divided into sequential subarrays comprising three adjacent fingers. The predicted binding interaction for each subarray was calculated against all possible 10-bp DNA sequences using a support vector machine [12] . The top 250 DNA sequences with the highest predicted binding potential for each subarray were then used to generate a nucleotide position weight matrix and position weight matrices from adjacent subarrays were merged assuming equal weight at overlapping positions. Sequence logo plots were then generated using ggPlot and seqLogo. Generation of the PRDM9 ZF phylogeny To make a comprehensive data set of known primate PRDM9 ZF sequences, we combined the ZFs sequenced in our study with those from refs 9 , 10 , 18 . Next, we removed the hypervariable nucleotide positions encoding DNA contact loci from the ZF sequences to limit noise during phylogenetic reconstruction. A multiple sequence alignment was then created (Clustal Omega) [26] and used to generate a maximum-likelihood tree with Phyml 3.0 (ref. 28 ). Approximate likelihood ratio tests above 0.8 are considered confident [28] , and we chose this as a threshold for marking branches with ‘strong’ support. FigTree was used for generating a graphical view of the phylogeny [29] . Accession codes: The DNA sequences generated in this study have been deposited in GenBank nucleotide database under the accession codes KJ916126 to KJ916191 . How to cite this article: Schwartz, J. J. et al. Primate evolution of the recombination regulator PRDM9. Nat. Commun. 5:4370 doi: 10.1038/ncomms5370 (2014).